A speciation gene for left–right reversal in snails results in anti-predator adaptation How speciation genes can spread in a population is poorly understood. In land snails, a single gene for left–right reversal could be responsible for instant speciation, because dextral and sinistral snails have difficulty in mating. However, the traditional two-locus speciation model predicts that a mating disadvantage for the reversal should counteract this speciation. In this study, we show that specialized snake predation of the dextral majority drives prey speciation by reversal. Our experiments demonstrate that sinistral Satsuma snails (Stylommatophora: Camaenidae) survive predation by Pareas iwasakii (Colubroidea: Pareatidae). Worldwide biogeography reveals that stylommatophoran snail speciation by reversal has been accelerated in the range of pareatid snakes, especially in snails that gain stronger anti-snake defense and reproductive isolation from dextrals by sinistrality. Molecular phylogeny of Satsuma snails further provides intriguing evidence of repetitive speciation under snake predation. Our study demonstrates that a speciation gene can be fixed in populations by positive pleiotropic effects on survival. Speciation occurs when populations accumulate genetic differences that, upon secondary contact, cause reproductive incompatibily [1] . How genes for reproductive incompatibilities (speciation genes) could spread in a population however, has been only poorly understood [2] , [3] , [4] . In land snails, instant speciation may occur once a population becomes fixed for left–right reversal by a single gene. Copulation between dextral (clockwise coiled) and sinistral (counterclockwise coiled) snails is usually strongly impeded by genital and behavioural mismatches, because they are reversed in genital position on the body side as well as in coiling direction [5] , [6] , [7] . The reversal is determined by a maternal effect of a single nuclear gene in at least four phylogenetically segregated families of pulmonate snails [6] , [8] , [9] , [10] . Thus, fixation for a reversal allele in an initially spatially isolated population could complete premating isolation between dextral and sinistral populations, giving rise to a new species [6] , [7] , [11] , [12] , [13] . In fact, left–right reversal has evolved many times, especially in terrestrial snails [14] , [15] . However, positive frequency-dependent selection resulting from difficulties of mating with the majority coiling phenotype is expected to eliminate the derived phenotype with reversed chirality [5] , [16] . Thus, as the two-locus model [17] , [18] , [19] predicts, speciation caused by a reproductive incompatibility at a single locus should only rarely proceed, without either genetic drift [11] , [13] or natural selection for the reversal that more than offsets the mating disadvantage [12] , [20] . Therefore, the origins of reversed snails have been puzzling. Southeast Asian snakes in the family Pareatidae are regarded as dietary specialists of terrestrial snails and slugs [21] ( Fig. 1a ). Because of the overwhelming predominance of dextral snails [14] , most pareatid snakes have evolved outstanding asymmetry in mandibular tooth number ( Fig. 1b ), which probably facilitates feeding on dextral snails [22] . The Japanese pareatid, P iwasakii , strikes an exposed soft part of a crawling snail from behind at a determined leftward angle to grasp the ventral shell surface with the upper jaw and the soft body by inserting the mandibles into the aperture. The snake then extracts the soft body by alternately protracting and retracting the asymmetric right and left mandibles ( Supplementary Movie 1 ). Because of this 'right handedness' of sequential behaviour, the snake can rarely grasp a sinistral snail ( Supplementary Movie 2 ). This survival advantage of sinistral variants may more than offset the mating disadvantage in dextral species and enhance the chance of population fixation for left–right reversal, which completes premating isolation [22] . 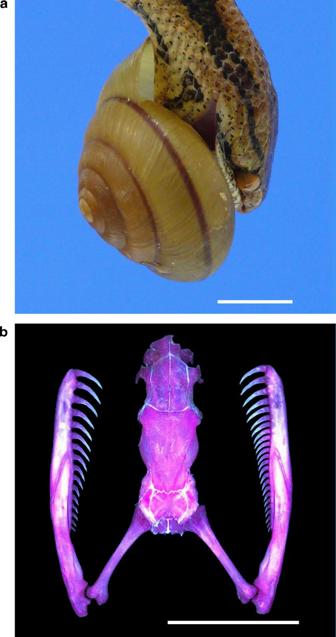Figure 1: The snail-eating snakeP. iwasakii. (a) Feeding behaviour ofP. iwasakii. (b) A skull specimen (dorsal view) ofP. iwasakii, exhibiting half a dozen more teeth on the right side of mandibles than on the left before hatching22,55. Bars: 10 mm. Figure 1: The snail-eating snake P. iwasakii . ( a ) Feeding behaviour of P. iwasakii . ( b ) A skull specimen (dorsal view) of P. iwasakii , exhibiting half a dozen more teeth on the right side of mandibles than on the left before hatching [22] , [55] . Bars: 10 mm. Full size image Our hypothesis predicts that sinistral lineages of snails more frequently emerge in sympatry with the snakes than in allopatry. Furthermore, the effect of snake predation on the emergence of sinistral lineages should be larger in groups of flat and/or large species for the following reasons. First, interchiral mating is almost impossible in flat snails which generally perform two-way face-to-face copulation, whereas it is relatively easy for tall snails which copulate by shell mounting [5] , [6] , [7] , [16] . Thus, populations are less likely to be fixed for the reversal solely by genetic drift in flat snails than in tall snails [5] , [13] . Second, snakes are generally gape limited [21] , and pareatid snakes cannot even hold a sinistral snail to prey upon unless the shell aperture is small enough [22] ( Supplementary Movie 2 ). Thus, the relative advantage of sinistrality under snake predation should also be larger in species with larger shells. Here, we tested these predictions by worldwide analyses of distributions of dextral and sinistral stylommatophoran snails and pareatid snakes. Furthermore, we examined the possible role of snake predation in the evolution of multiple sinistral lineages by the analyses of molecular phylogeny and biogeography of snails in the genus Satsuma . This study illustrates how a single gene for reproductive incompatibility could generate a new species by natural selection for ecological adaptation. Feeding experiments In our experiments with dextral and sinistral Satsuma species, none of the dextral snails survived snake predation ( Fig. 2 ; Supplementary Movie 1 ). In strong contrast, 87.5% of the sinistral snails survived predation ( Supplementary Movie 2 ). The interaction effect of coiling direction and shell size on survival was significant (likelihood ratio test (LRT) for comparing generalized linear mixed models (GLMMs), d.f.=1, χ 2 =10.8, P <0.01; Fig. 2 ) when the effects of snake individual and snail groups were statistically removed in the combined data set including the results of the study by Hoso et al . [22] This analysis, however, did not exclude the effects of interspecific differences in characteristics other than coiling direction, which potentially influence the survival rate. Throughout the experiment, snakes did not change the right-handed attacking behaviour. Snail extraction has commonly been observed in six other pareatid species ( Aplopeltura boa , P. boulengeri , P. carinatus , P. formosensis , P. margaritophorus and P. stanleyi ). 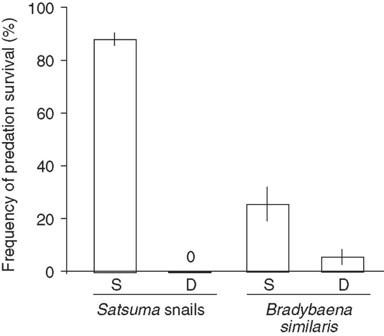Figure 2: Survival advantage of sinistral snails. Each bar indicates the proportion of successful survival of sinistralS. perversaand dextralS. mercatoria(left), and of sinistral variant and dextral wild-typeB. similaris(right) against predation byP. iwasakii(means across four snakes±s.e.;n=10 for each snake). S indicates attempts on sinistrals and D on dextrals. Figure 2: Survival advantage of sinistral snails. Each bar indicates the proportion of successful survival of sinistral S. perversa and dextral S. mercatoria (left), and of sinistral variant and dextral wild-type B. similaris (right) against predation by P. iwasakii (means across four snakes±s.e. ; n =10 for each snake). S indicates attempts on sinistrals and D on dextrals. Full size image This advantage of sinistrality results from a mechanical mismatch between the snake's right-handed predation behaviour and the snail's left-handed coiling structure. The snake does not modify the right-handed attacking behaviour. Thus, to hold a sinistral snail, the snake must reach the upper jaw onto the dorsal shell surface across the aperture, while inserting the lower mandibles under the soft body. However, due to the gape limitation [21] , the snake can hardly achieve it when the snail's aperture is relatively large. For this reason, the survival advantage of sinistrality was much larger in snails of the genus Satsuma compared with Bradybaena similaris . Thus, the result of our feeding experiment suggests that the survival advantage of sinistrality varies depending on the shell size, and thus the evolution of sinistral species in response to the right-handed predation by pareatid snakes may be more frequent in groups of larger snails. Comparative survey We found that sinistral genera are marginally associated with snail-eating pareatid snakes in geographical distribution ( Table 1 ; LRT for comparing GLMMs, d.f.=1, χ 2 =5.5, P =0.019). The statistical test incorporating distribution, shape and their interaction indicated that sinistral genera are more strongly associated with the sympatry with the snakes in flat snails than that in tall snails (LRT for comparing GLMMs, d.f.=1, χ 2 =9.8, P <0.01; Fig. 3a,b ). The effect of interaction between distribution and size was also significant (LRT for comparing GLMMs, d.f.=1, χ 2 =8.6, P <0.01; Fig. 3c ). Thus, the association of sinistral genera with the snakes is stronger in flat snails than in tall snails and larger snails. These findings cannot be explained by a phylogenetic artifact because the effect of higher taxa was statistically removed in every analysis by incorporating higher taxa (family) as a random effect ( Fig. 4 ). Table 1 Association of geographical distributions between sinistral land snails and pareatid snakes. 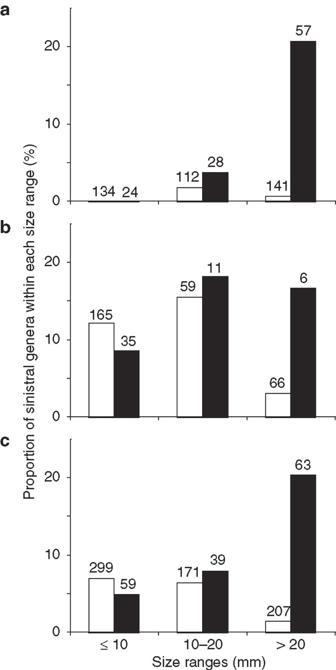Figure 3: Shell-size-dependent associations of distributions between sinistral land snails and pareatids. Each bar indicates the proportion of genera composed of sinistral species in a 10-mm shell diameter interval ((a), flat snails; (b), tall snails; (c), total) showing the outcome of statistical analyses that used individual shell sizes as a numerical variable. Closed and open bars indicate the proportions within and outside the range of pareatid snakes, respectively. The number above each bar indicates the total number of genera included in each size range. Full size table Figure 3: Shell-size-dependent associations of distributions between sinistral land snails and pareatids. Each bar indicates the proportion of genera composed of sinistral species in a 10-mm shell diameter interval (( a ), flat snails; ( b ), tall snails; ( c ), total) showing the outcome of statistical analyses that used individual shell sizes as a numerical variable. Closed and open bars indicate the proportions within and outside the range of pareatid snakes, respectively. The number above each bar indicates the total number of genera included in each size range. 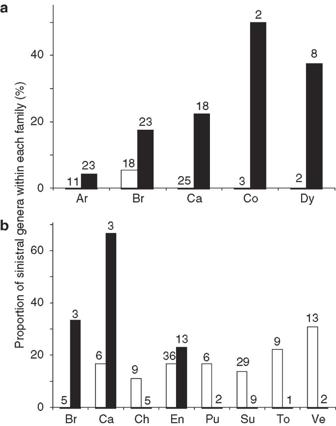Figure 4: Taxon-independent association of distributions between sinistral land snails and pareatid snakes. Each bar indicates the proportion of genera composed of sinistral (a) flat-shelled and (b) tall-shelled species. Closed and open bars indicate the proportions within and outside the range of pareatid snakes, respectively. Family names are denoted by the following abbreviations; Ariophantidae (Ar), Bradybaenidae (Br), Camaenidae (Ca), Chondrinidae (Ch), Corillidae (Co), Enidae (En), Dyakidae (Dy), Pupillidae (Pu), Subulinidae (Su), Tornatellinidae (To) and Vertiginidae (Ve). Families distributed across both ranges are shown. The number above each bar indicates the number of genera included in each family. Full size image Figure 4: Taxon-independent association of distributions between sinistral land snails and pareatid snakes. Each bar indicates the proportion of genera composed of sinistral ( a ) flat-shelled and ( b ) tall-shelled species. Closed and open bars indicate the proportions within and outside the range of pareatid snakes, respectively. Family names are denoted by the following abbreviations; Ariophantidae (Ar), Bradybaenidae (Br), Camaenidae (Ca), Chondrinidae (Ch), Corillidae (Co), Enidae (En), Dyakidae (Dy), Pupillidae (Pu), Subulinidae (Su), Tornatellinidae (To) and Vertiginidae (Ve). Families distributed across both ranges are shown. The number above each bar indicates the number of genera included in each family. Full size image In a LRT between generalized linear models (GLMs) that accounts for shell sizes of dextral and sinistral congeners (33 genera), the interaction of the effect of snakes and coiling direction on shell size was not significant (LRT for comparing GLMs, χ 2 =0.126, d.f.=1, P =0.723). This suggests that snake predation is not likely to be responsible for the shell size of sinistral snails. Phylogenetic analyses In our phylogenetic analyses of the snail genus Satsuma in Japan and Taiwan ( Fig. 5a ), the combined data matrix consisted of 2,842 nucleotide sites, of which 779 were parsimony informative. The maximum parsimony (MP) analysis resulted in the two most parsimonious trees (5,337 steps, consistency index excluding uninformative characters=0.2631, retention index=0.6068). The result of maximum likelihood (ML) and Bayesian analyses were largely consistent with the result of the MP analysis ( Fig. 5b , Supplementary Fig. S1 ). In both the combined and separate data sets, the likelihood values of the constrained trees for sinistral lineage to be monophyletic were significantly lower than those of the unconstrained best trees (the approximately unbiased (AU) test [23] , [24] , all P -values <0.01), indicating that the sinistral species have evolved from dextral ancestors multiple times within Satsuma . 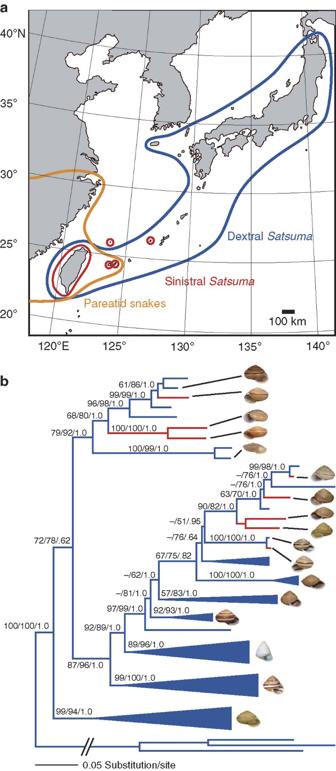Figure 5: Distribution and phylogeny of the snail genusSatsuma. (a) Geographical distributions of sinistral (red) and dextral (blue) snails and pareatid snakes (orange) in East Asia. (b) Phylogenetic relationships of sinistral (red) and dextral (blue) snails based on maximum likelihood analysis of the combinedCO1,ITSandETSsequence data. Several clades containing only dextral species are compressed in blue (seeSupplementary Fig. S1for details). Specific names are listed inSupplementary Data 2. The numbers on branches indicate MP and ML bootstrap values, followed by Bayesian posterior probabilities (<50% not shown). Shells of some representative species are shown. Figure 5: Distribution and phylogeny of the snail genus Satsuma . ( a ) Geographical distributions of sinistral (red) and dextral (blue) snails and pareatid snakes (orange) in East Asia. ( b ) Phylogenetic relationships of sinistral (red) and dextral (blue) snails based on maximum likelihood analysis of the combined CO1 , ITS and ETS sequence data. Several clades containing only dextral species are compressed in blue (see Supplementary Fig. S1 for details). Specific names are listed in Supplementary Data 2 . The numbers on branches indicate MP and ML bootstrap values, followed by Bayesian posterior probabilities (<50% not shown). Shells of some representative species are shown. Full size image The results of feeding experiments support our hypothesis that under 'right-handed' predation by pareatid snakes, the survival advantage of sinistral variants may counterbalance their mating disadvantage. In this case, selective predation may facilitate population fixation for the sinistral allele and simultaneously cause speciation. This hypothesis predicts that the diversity of sinistral taxa is higher in the range of the snail-eating snakes. Our biogeographical analyses supported this prediction. Pareatid snakes may have continued specialized predation since their early phylogenetic segregation in the Colubroidea [22] , [25] . No terrestrial snail predators other than the snakes are known to specialize for prey handedness [26] . Therefore, our results are consistent with the hypothesis that 'right-handed' snake predation drives snail speciation by left–right reversal. Further experimental studies may be desired to examine the effect of shell shape on the snake's predation success [27] . The analysis of phylogeny was necessary to distinguish speciation by reversal from monophyletic diversification of sinistrals. However, no phylogenetic hypothesis of snail taxa in a global scale has been available. As a test case, we examined the molecular phylogeny of the genus Satsuma , which includes multiple dextral and sinistral species in the snake range. In natural conditions, P. iwasakii preys on dextral species of Satsuma [28] , which exhibit defensive aperture morphology against snake predation [27] . Thus, Satsuma snails have probably been subject to severe snake predation. Superiority of sinistral Satsuma species in our feeding experiments suggests that the phylogeny of Satsuma may reflect the history of prey–predator interactions with the snakes. The presence of multiple sinistral Satsuma lineages within the monophyletic genus can hardly be explained by introgression via hybridization with dextral snails after completion of speciation, because Satsuma snails perform face-to-face copulation that prevents interchiral mating [5] . Thus, these sinistrals must have evolved in one of three possible scenarios: independent fixation for sinistrality in each lineage, a single event of fixation for a sinistrality that temporally represents ancestral polymorphism or combination of these. Fixation for sinistrality should be rapid because both directional selection by snake predation and positive frequency-dependent selection cooperate for sinistrality once sinistral variants become more common than dextrals under the snake predation, while other populations of the ancestral species remain dextral. Consequently, a sinistral species could be composed of non-sibling populations unless lineage sorting is complete, as seen in the polyphyletic mitochondrial lineages of a dextral species derived from a sinistral Euhadra species outside the range of pareatid snakes [20] . In contrast, our multilocus analyses strongly supported the independent origins of sinistral Satsuma by deep branching into three clades. Overall, our results suggest that the mating disadvantage of left–right reversal has independently been resolved in the multiple sinistral lineages. These events of evolution to sinistrals may be too frequent in such a narrow geographical range to attribute to fixations solely by genetic drift. The virtual absence of sinistral Satsuma outside the range of pareatid snakes supports the likelihood that left–right reversal is higher under predation by the snakes. Relatively recent repetition of emergence of a sinistral lineage also suggests that right-handed predation by the snakes may also currently be creating new sinistral species by left–right reversal in Satsuma . However, our result does not rule out the possibility that the proportion of sinistral taxa per lineage might have apparently been amplified by extinctions of dextral taxa because of snake predation. The presence of sinistral genera outside the snake range indicates that sinistral species have also evolved without snake predation, for example, resulting from reproductive characteristic displacement [20] , [29] , [30] , or stochastic fluctuation [6] . These events should be as frequent in sympatry with the snail-eating snakes as in allopatry. Thus, we do not conclude that snake predation is responsible for the origin of every sinistral snail species inside the snake ranges. One primary prey for a snake predator disappears through each event of population fixation for reversal. Local accumulation of sinistral snails may eventually diminish the advantage of right handedness for the snake and prompt the counteradaptive evolution of 'left-handed' snakes, just as the handedness ratio oscillates in scale-eating cichlid fishes [31] . However, pareatid snakes with reversed dentition have never been found across Southeast Asia [22] . Yet, dextral snails remain the majority at genus level and predominant in the snake range. Indeed, dextral snails available for P. iwasakii are not only species-rich but also still abundant in snail communities [28] . Thus, the snakes could have shifted prey to less-protected alternatives and enjoyed the advantage of right handedness, as theories of optimal foraging and coevolutionary alternations [32] , [33] predict. These ecological differences between predator snakes and prey snails may underlie the absence of counteradaptive responses by pareatid snakes, allowing the prey to repeat evolutionary escape by speciation. Generally, identification of an isolation barrier that initiated speciation is rarely possible because subsequent genetic and ecological divergence builds up additional barriers that confound analysis [34] , [35] , [36] , [37] . However, instant speciation of snails by left–right reversal is exceptional [34] , where the speciation gene may hardly change ecological features, such as resource use or habitat preference, except for susceptibility to snake predation and partners to mate. In the secondary contact with a new sinistral population (species), dextral ancestors without additional ecological divergence would go extinct because of a severe survival disadvantage under snake predation. Thus, not only reversal but also other mechanisms are required for the coexistence of dextral and sinistral congeners in Satsuma . Their coexistence may offer rare opportunities to distinguish post-speciation divergences from the cause of speciation, bridging our understandings of speciation and community assembly. Our study demonstrated how positive selection could operate for major pleiotropic effects of a speciation gene on anti-predator survival, exemplifying a 'magic trait' [38] that simultaneously gives rise to adaptation and reproductive isolation. Speciation by natural selection may initially require genetically simpler changes of phenotype than previously expected. Our evidence for the evolutionary role of single-gene pleiotropy resurrects Goldschmidt's controversial idea of hopeful monsters [39] . Feeding experiments We conducted predation experiments between August 2004 and August 2005 at Kyoto University in accordance with the Institutional Regulation on Animal Experimentation. As predator snakes, we used four individuals of P. iwasakii (three from Ishigaki Island and one from Iriomote Island; snout-vent length: 430–580 mm; head width: 7.6–9.5 mm; two of the snakes were also used in the study by Hoso et al . [22] ). As prey snails, we used snails from the genus Satsuma : S. mercatoria (dextral) in Okinawa Island and S. perversa (sinistral) in Kume Island, the Ryukyu Archipelago, Japan. Satsuma snails (mean±s.d.=27.4±1.9 mm in shell diameter) were larger than B. similaris (12.7±1.5 mm) used in the study by Hoso et al . [22] S. mercatoria and S. perversa are suitable for this study, because they resemble each other in shape and size and are closely related ( Fig. 5b ). To exclude the potential effects of local adaptation and learning by predators and prey, we collected these snails from islands where no pareatid snakes occur. To test the interactive effect of sinistrality and size of snails on survival rate from snake predation, we performed LRTs between null models and test models where the focal factor was additionally incorporated as a fixed effect. As covariates, we adopted coiling direction, shell diameter and snail groups ( Satsuma spp. or B. similaris ). We incorporated snake individuals as random effects to avoid pseudo-replication resulting from using the same snakes repeatedly. Comparative survey We classified all of the recent terrestrial snail genera of the order Stylommatophora by size, shape, coiling direction and distribution according to the information available in the literature ( Supplementary Information ). We excluded taxa unsuitable for the analysis, that is, slugs with no or reduced shells, species that are chirally dimorphic in 11 genera [5] and the sinistral superfamily Clausilioidea, for the following reasons. Slug and chirally dimorphic taxa do not fit binary classification by coiling direction. Inclusion of the latter did not affect the result. The Clausilioidea is a cosmopolitan monophyletic taxon with a few exceptional dextral lineages, which is most likely to descend from the single sinistral ancestor. Thus, they do not provide meaningful values to test the distribution of reversal events from the dextral to the sinistral. Although it might be of use for the examination of opposite reversal from the sinistral to the dextral, it is irrelevant to the purpose of the present study. In this paper, we call a genus including sinistral species as a sinistral genus. Sympatric genera means that they are partly or fully sympatric with snail-eating pareatid snakes. In binary classification of genera, we treated 33 genera that include both dextral and sinistral species as the indication of separate reversal events. As the shell size of each genus, we used the shell diameter of the largest species in the genus because it was the only size indicator listed in every literature we referred. Shell diameter was log-transformed for the following parametric analysis. Bimodal shell shapes are associated with discrete mating behaviours; tall-shelled snails usually mate by shell mounting, and globular- to flat-shelled snails mate face-to-face [5] , [40] albeit with several exceptions [41] . Probably because interchiral mating is physically easier and thus positive frequency-dependent selection is relaxed in species with shell-mounting copulation, sinistral genera have more frequently evolved in tall-shell shaped taxa in pulmonates [5] , [7] . Therefore, the shell shape may generate potentially important covariance in the test of our hypothesis. Tall genera were defined as having the shell height greater than the shell diameter, globular to flat genera as having the height equal to or less than the diameter. This simple definition reflects the bimodality in the shell shape of terrestrial stylommatophoran pulmonates, as originally reported by Cain [42] and subsequently by others (for example, ref. 43 ). Genera were assigned to two degrees at ordinal scales; 342 tall genera into 1, and 485 flat genera and 11 genera containing both tall and flat species into 0. The examined data matrix is provided in Supplementary Data 1 . To test the effects of snakes (sympatry or allopatry with pareatid snakes; test 1), interaction between snakes and size (maximum shell-diameter; test 2) and interaction between snakes and shape (tall or flat-shell shape), on the occurrence of sinistral genera (test 3), we separately performed LRTs between null models and test models where each focal factor was additionally incorporated as a fixed effect. As covariates, we adopted size and shape for test 1, and snakes, size and shape for test 2 and test 3. We incorporated the family to which each snail genus belongs as a random factor to avoid the potential bias due to the increase of sinistral genera by monophyletic radiation. Because multiple families include sinistral genera regardless of shell shape ( Fig. 4 ), local distributions of particular snail taxa did not affect our global scale analysis. Additionally, we tested an alternative hypothesis that snake predation favours the evolution of larger shells in sinistral snails instead of that of sinistrality in larger dextral snails. We analysed the data using R version 2.11.1 in Windows [44] with the lme4 and glm packages. The summaries of analyses are provided in Supplementary Table S1 . Molecular methods To reconstruct a species level phylogeny, we sampled 75 species of Satsuma , including all species that inhabit the Ryukyu Archipelago except a sinistral species ( S. tadai ) endemic to Uotsuri Island ( Supplementary Data 2 ). We sequenced partial regions of mitochondrial cytochrome b oxidase subunit 1 gene ( CO1 ) and nuclear ribosomal external transcribed spacer ( ETS ) and complete sequence of nuclear ribosomal internal transcribed spacers ( ITS ) 1 and 2. DNA extraction, PCR amplification, and sequencing of CO1 and ITS were performed following the previously described method [45] . PCR amplification of ETS fragment was performed using primers Satsuma-ETSf (5′-CTCCAGCCCGGCGTWTGGCG-3′) and 18Sop (5′-GCTCCCTCTCCGGAATCGAACCC-3′) under the following conditions: initial denaturation for 3 min at 94°C, followed by 30 cycles of 30 s at 94°C and 1 min at 72°C, with a final extension for 3 min at 72°C. Sequencing of ETS region was performed using primers Satsuma-ETSf and Satsuma-ETSr (5′-TTTAATGAGCCATTCGCGG-3′). The obtained sequence data have been uploaded to GenBank and the accession codes are provided in Supplementary Data 2 . Phylogenetic analyses Alignment of the CO1 sequences was straightforward with no gaps. ITS and ETS sequences were aligned using ClustalX [46] with manual adjustments. Gaps were treated as missing data. For outgroups, we used three camaenid species, Nipponochloritis hiromitadae , N. oscitans iwatensis and Yakuchloritis albolabris . We conducted phylogenetic analyses of the combined data of three genes based on the MP, ML and Bayesian methods. MP analyses were performed using PAUP* 4.0b10 [47] . We performed heuristic searches with ten random additional analyses and tree bisection-reconnection (TBR) branch swapping. The resulted trees were used as starting trees in an additional round of heuristic search with TBR branch swapping. Bootstrap analysis was performed based on 1,000 replicates of heuristic searches with ten random addition analyses and TBR branch swapping, saving no more than 100 trees per analysis. Before the ML and Bayesian analyses, we determined an appropriate model of sequence evolution and model parameters using Kakusan version 3.0 [48] . ML analyses were performed using Treefinder [49] with the 100 iterations of the likelihood ratchet implemented in Phylogears [50] . Bootstrap analysis was conducted based on 1,000 replications. Bayesian analyses were performed using MrBayes v3.1.2 [51] . The analysis was carried out by two simultaneous runs, each of which consisted of running four simultaneous chains for six million generations and sampling trees every 1,000 generations. We discarded first 1,501 trees as burn-in, and the remaining 9,000 samples were used to estimate the tree topology, branch length, and substitution parameters. We tested the hypothesis of the monophyly of the sinistral Satsuma lineages by the AU test [23] , [24] for both combined and separate data sets of the three genes. The alternative trees were obtained by ML heuristic search as described above under the topological constraint (sinistral lineage monophyletic), and the AU test was conducted based on 1,000,000 replications using Treefinder [49] . A phylogenetically informed test for the independence of two characters [52] cannot be adequately performed in this case, because the absence of the snakes does not favor the evolution of dextral snails by left–right reversal, and their presence does not always result in the evolution of sinistral snails. Our hypothesis predicts the different rates of character transition in snail coiling between clades depending on whether they have been under snake predation or not. In this case, maximum likelihood estimation of ancestral traits is not reliable, because it assumes the equal character-transition rates across all the clades. To avoid this artefact, we estimated ancestral states based on the most parsimonious scenarios. Although we independently reconstructed ancestral character states based on ML and Bayesian methods as implemented in BayesTraits [53] for a clade including 37 OTUs (operational taxonomic units; listed at the top of Supplementary Data 2 ) completely coexisting with the snakes, the probabilities of sinistral state in the best models converged around 0.5 at most nodes. Reconstructing the ancestral state of a functional trait that is subjected to stringent natural selection requires a caution as follows. If the directional selection for sinistrality continues for a long time, the proportion of dextral lineages may decrease, and thus the phylogeny inferred for extant species may underestimate the number of reversals to sinistrality. Thus, our result may have underestimated the frequency of reversal in snails because of using a genus or monophyletic lineage as a unit to count. This shortcoming is inevitable unless the entire evolutionary history in question could be recovered [54] . How to cite this article: Hoso, M. et al . A speciation gene for left-right reversal in snails results in anti-predator adaptation. Nat. Commun. 1:133 doi: 10.1038/ncomms1133 (2010).